Diffusion on networked systems is a question of time or structure Network science investigates the architecture of complex systems to understand their functional and dynamical properties. Structural patterns such as communities shape diffusive processes on networks. However, these results hold under the strong assumption that networks are static entities where temporal aspects can be neglected. Here we propose a generalized formalism for linear dynamics on complex networks, able to incorporate statistical properties of the timings at which events occur. We show that the diffusion dynamics is affected by the network community structure and by the temporal properties of waiting times between events. We identify the main mechanism—network structure, burstiness or fat tails of waiting times—determining the relaxation times of stochastic processes on temporal networks, in the absence of temporal–structure correlations. We identify situations when fine-scale structure can be discarded from the description of the dynamics or, conversely, when a fully detailed model is required due to temporal heterogeneities. The relation between network structure and dynamics has attracted the attention of researchers from different disciplines over the years [1] , [2] , [3] , [4] , [5] . These works are rooted in the observation that in contexts as diverse as the Internet, society and biology, networks tend to possess complex patterns of connectivity, with a significant level of heterogeneity [4] . In addition, a broad range of real-world dynamical processes, from information to virus spreading, is akin to diffusion. If the effect of structure, such as communities or degree heterogeneity, on diffusive processes is now well known [6] , [7] , the impact of the temporal properties of individual nodes is poorly understood [1] , [8] . Yet, empirical evidence indicates that real-world networked systems are often characterized by complex temporal patterns of activity, including a fat-tailed distribution of times [9] , [10] , [11] , [12] , [13] , [14] , [15] , [16] , correlations between events [17] , [18] and non-stationarity [19] , [20] , [21] . This is in remarkable contrast to a vast majority of mathematical models, which assume homogeneous interaction dynamics on networks [1] , [2] , [22] , [23] . In this work, we focus on the impact of structure and the waiting-time distribution on dynamics, and set aside any other temporal properties. This subject has triggered intense theoretical work in recent years, for example, in relation to anomalous diffusion, but predominantly on lattice-like, annealed [24] and random structures [20] , [23] , [25] , [26] , [27] , [28] . These limitations leave a fundamental question open, with important applications for the modelling of temporal networks: what are the effects of complex patterns, simultaneously in time and in structure, on the approach to equilibrium of diffusion processes? To comprehend the interplay between temporal and structural patterns, we focus on a broad class of linear multi-agent systems describing N interacting nodes, defined by where x i , the i th component of x , represents the observed state of node i . The N × N real matrix L encodes the mutual influences in the network, with non-zero entries indicating the presence of a link. D is either d/d t , the delay Dx i ( t )= x i ( t +1), or any other causal operator acting linearly on the trajectory of each entry x i ( t ). This equation couples network structure (represented by L ) and time evolution (represented by D ) by describing a system where every node i has a state x i ( t )= Fu i ( t ), where u i ( t )=Σ j L ij x j ( t ) represents the input, or influence of the neighbouring states on node i . The operator F is the so-called transfer function [29] , [30] , defined as the inverse of D (see Methods). A classic example is heat diffusion on networks, where every node has a temperature x i evolving according to the Fourier Law where μ is the characteristic time of the dynamics and L is a Laplacian of the network. The same set of equations can represent, possibly up to a change of variables, a basic model for the evolution of people’s opinions [31] , robots’ positions in the physical space [30] , [32] , approach to synchronization [33] , [34] or the dynamics of a continuous-time random walker [35] —our main example from now. In any case, the dynamical properties of the system are described by the spectral properties of the coupling matrix. The constraints imposed by the conservation of probability imply that the Laplacian dynamics is characterized by a stationary state, associated to the dominant eigenvector of L , which we will assume to be unique, as is the case in a large class of systems, for example, strongly connected networks. A key quantity is thus the second dominant eigenvalue, also called the spectral gap [6] , which provides us with the relaxation time to stationarity, usually called mixing time [36] for stochastic diffusion processes. The spectral gap determines the speed of convergence to the stationary state and measures the effective size of the system in terms of dynamics. The spectral gap is also related to important structural and dynamical properties of the system, such as the existence of bottlenecks and communities in the underlying network [7] , [30] . In this study, we generalize the concept of spectral gap and of mixing time to random processes with general causal operator D , and focus in detail on operators with long-term memory, naturally emerging in diffusion with bursty dynamics. After showing connections between the theory of random walks and that of multi-agents systems, we identify the temporal and structural mechanisms driving the asymptotic dynamics of the system and provide examples when each mechanism prevails. By doing so, we show that the form of the temporal operator D may either slow down or accelerate mixing as compared with the differential operator equation (2). The results are further exploited to assess the possibility of coarse-graining the dynamics based on the network community structure and tested using numerical simulations on synthetic temporal networks calibrated with empirical data. Random walks with arbitrary waiting times The generalized dynamics of the random walker, illustrated in Fig. 1a , is defined as follows. A walker arriving at a node i jumps towards a neighbouring node within a time interval [Δ t ,Δ t+δ ] with probability ρ (Δ t ) δ (for small δ ). In line with a standard discrete-time random walk process, the jump is directed towards a neighbour j with probability P ij . The probability density function ρ (Δ t ) is called the waiting- time distribution of the walker. At each hop, the waiting time Δ t is reset to zero and consecutive waiting times are independent. The evolution of probability of the presence of a stochastic process in each state is ruled by the so-called master equation, or Kolmogorov forward equation, well known for this family of generalized walks [24] , [37] , [38] . We prefer to adopt here the equivalent, dual, viewpoint of Kolmogorov backward equation [39] , which belongs to the class of processes defined by equation (1) and can be analysed using the toolbox typical to multi-agent systems [30] , [32] , such as the transfer function formalism and eigenmode decomposition. 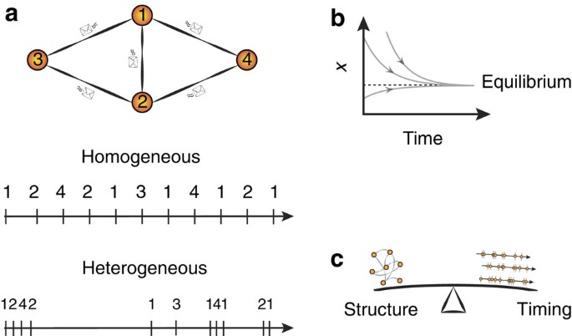Figure 1: Diffusion on temporal networks. (a) A random walk process can be illustrated by a letter (or banknote and so on) being randomly passed from neighbour to neighbour on a social network. Temporal patterns of waiting times between arrival and departure of the letter may be homogeneous (for instance, discrete or exponentially distributed times) or heterogeneous (for instance, bursts). (b) The relaxation time measures the characteristic time to reach equilibrium from any starting condition. (c) The competition between structure and temporal patterns regulates the relaxation time, or mixing time, of stochastic processes. Figure 1: Diffusion on temporal networks. ( a ) A random walk process can be illustrated by a letter (or banknote and so on) being randomly passed from neighbour to neighbour on a social network. Temporal patterns of waiting times between arrival and departure of the letter may be homogeneous (for instance, discrete or exponentially distributed times) or heterogeneous (for instance, bursts). ( b ) The relaxation time measures the characteristic time to reach equilibrium from any starting condition. ( c ) The competition between structure and temporal patterns regulates the relaxation time, or mixing time, of stochastic processes. Full size image We assign a fixed real-valued observable x obs ,i to every node i and consider the value observed at time t by a walker starting initially from node j . This value is a random variable, with an expected value denoted by x j ( t ), taking initial value x j (0)= x obs ,j . The random walk is ergodic and mixing on a strongly connected aperiodic network (aperiodicity is only required for the discrete time, when ρ (Δ t ) is a Dirac distribution). In this case, x ( t ) describes a consensus dynamics, meaning that the individual values asymptotically converge to one another, x i (∞)= x j (∞). If we choose the observable x obs ,j =0 at all nodes j , except l at node k , then x i ( t ) is precisely the probability for the random walker starting at i to be found at k at time t . Therefore, the Kolmogorov backward equation, a consensus dynamics, embeds in particular the evolution of the probability of the presence on nodes. The walker, assumed to have just hopped at time zero and finding itself at node i (another origin of time would not change the asymptotic decay times, of main interest in this work), hops again at time Δ t with probability density ρ (Δ t ) and moves towards a neighbour j with probability P ij . The expected value observed by the walker at time t is x obs ,i if it is still waiting for its first hop ( t <Δ t ) and otherwise Σ j P ij x j ( t −Δ t ), by induction on the number of hops. Therefore, we obtain the vector equation with the discrete transition matrix P of entries P ij . The convolution in time in the last term calls for a Laplace transform For simplicity, we use the same notations for functions in the time and in the Laplace domain, only distinguished by their variable, namely t or Δ t for time and s for Laplace. This is justified as time and Laplace domain representations encode the same single physical object, for example, a probability or an observable. The same holds for operator D , thought of as acting in the time domain (for instance D =d/d t ) or the Laplace domain ( D = s ) according to the context. The Laplace transform ρ ( s ) is the moment generating function of the waiting-time distribution ρ (Δ t ), as it encodes the moment in its Taylor series , where μ is the expected waiting time (first moment), σ 2 is the variance and μ 2 + σ 2 is the second moment. Using the fact that convolution (respectively, integration from 0 to t ) in the time domain corresponds to the usual product (respectively, division by s ) in the Laplace domain [40] , equation (3) reduces to or equivalently where we have made the dependence on the initial condition explicit by using the relation x obs = x ( t =0) and where L = P – I denotes the (normalized) Laplacian of the network. This is an instance of equation (1), which shows that an input–output relationship is often best expressed in the Laplace domain rather than in the temporal domain. In this case, the transfer function F ( s ) is defined by the algebraic relation F −1 ( s )=1/ ρ ( s )−1= D ( s ), up to the initial condition term, implicit in equation (1). See Methods for a derivation of equation (1) in a more general context. From temporal networks to random walks Diffusive processes often take place on temporal networks where individuals initiate from time-to-time short-lived contacts with their neighbours. A random walker can represent, for example, a letter or a banknote passing from hand to hand through first contact initiated by the current node. The formalism described above focuses on the statistical properties of the waiting times of a walker on a node [15] , [25] , and not of the inter-contact times (the times between two subsequent contacts from a given node to another), as often considered in the literature [20] , [27] , [28] , [41] , [42] , [43] . To illustrate this difference, let us consider an idealized scenario, where the network looks locally similar to a directed tree, to avoid indirect correlations due to cycles [44] , where the inter-contact time t between two contacts initiated by the same node is characterized by the same probability distribution ρ contact ( t ), and where activations on different edges are an independent random process. The corresponding waiting-time distribution ρ (Δ t ) for the random walker can be determined from ρ contact [45] , [46] . For example, the classic inspection paradox, or bus paradox, observes that the waiting time has a mean which can be much higher than the average inter-contact time μ contact in case of bursts. This fact has been used in the literature to deduce that burst contact statistics slowdown diffusion in a complex network [43] . Nevertheless, it should not be confounded with the results presented in this paper, which will focus on the statistical properties of the waiting-time distribution and identify, among others, that its variance plays a significant role on the asymptotic behaviour of the walker. In the above scenario, the variance of ρ (Δ t ) depends on the third moment of the inter-contact time distribution ρ contact ( t ) and is associated to a mechanism distinct from that of the bus paradox (equation (7)). Eigenmodes for heterogeneous temporal operators Equation (1) typically takes the form of an integro-differential equation. However, it simplifies into the differential equation (2) in the case of a memoryless random walker. Memoryless refers to the case when the probability of hopping between Δ t and Δ t+δ , knowing that the walker has waited at least Δ t , is independent of Δ t . This leads to an exponential waiting-time distribution [45] ρ (Δ t )= e −Δ t/μ /μ , in other words an unconditional probability e −Δ t/μ δ / μ of jumping between Δ t and Δ t+δ , for small δ and for mean waiting time μ . In that case, we find D ( s )=1/ ρ (s)−1= μs in the Laplace domain, indeed recovering equation (2) in the time domain. The differential equation can then be analysed by changing the variables x to a linear combination of the eigenvectors v k of the Laplacian L , of eigenvalues λ 0 =0> λ 1 , λ 2 ,..., λ N −1 ≥−2 as follows [30] : For simplicity we have supposed that the underlying network is undirected, connected and, in case of a discrete-time random walk, non-bipartite. Thus, the eigenvalues are real and the stationary state is uniquely defined [6] . Every z k ( t ), solution of Dz k ( t )= λ k z k ( t ), is called an eigenfunction of the operator D and here takes the form of a decaying exponential. The problem is thus solved by decoupling structural and temporal variables, first by identifying structural eigenvectors ( v k ), and then how they evolve in time ( z k ( t )). The resulting fundamental solutions z k ( t ) v k for equation (1) are called modes, or eigenmodes, of the system. A similar analysis can be performed in the Laplace domain in the case of an arbitrary waiting-time distribution ρ (Δ t ), and thus when equation (1) has an arbitrary temporal operator D . In that case, the elementary solutions z k ( t ), associated to z k ( s ), need not be exponential functions and are obtained as solutions of equation (6), where the Laplacian is reduced to its eigenvalue λ k As before, any trajectory of the system can be expressed as a linear superposition of some or all the N modes. Characteristic decay times of eigenmodes Despite their non-exponential nature, a broad class of eigenfunctions defined by equation (9) still have a characteristic time τ k describing the asymptotic decay of z k ( t ) to equilibrium as ( Fig. 1b ). We find that the decay time can be accurately estimated by performing a small s expansion in the Laplace domain (see Methods for the derivation and range of validity): where is a measure of the burstiness of the temporal process based on the first and second moments of its distribution. Burstiness β equals to zero for a Poisson process (memoryless waiting times, ρ (Δ t )= e −Δ t / μ / μ ) and ranges from−1/2 (if ρ (Δ t ) is a Dirac distribution) to arbitrarily large positive values (for highly bursty activity). This expression emerges naturally from the dynamical process and can be viewed as a measure of burstiness, equivalent to the commonly used burstiness measure [47] . The estimate provided by equation (10) can be further tightened whenever the distribution ρ (Δ t ) of waiting times contains a fat tail, possibly softened by an exponential tail. The archetypical example is a power law with soft cutoff, , a frequent model in human dynamics supported by empirical evidence [9] , [14] , [41] . More generally, , where ρ 0 is a fat tailed distribution, that is, decreasing subexponentially. The non-analytic point created in ρ ( s ) by the fat tail leads to an additional term in the characteristic time (see Methods) which can be approximated as follows, if | λ k | −1 and β have different orders of magnitude Mixing times and dominating mechanisms Of particular importance is the slowest non-stationary mode ( k =1), or mixing mode, the characteristic decay time of which represents the worst-case relaxation time of any initial condition to stationarity. We call this time the mixing time of the process, in generalization of the classic memoryless case, where it is given by , determined by the so-called spectral gap (refs 6 , 36 ). This quantity is related to the presence of bottlenecks (that is, weak connections between groups of highly connected nodes, a.k.a. network communities) in the network (via Cheeger’s inequality [48] , [49] ). It is approximated as This expression shows that the asymptotic dynamics of each mode is determined by the competition between three factors: a structural factor associated to the spectral properties of the Laplacian of the underlying network and two temporal factors associated to the shape of the waiting-time distribution, namely its burstiness ( μβ ) and its exponential tail ( τ tail ). The slowest (largest) of these factors dominates the asymptotic dynamics ( Fig. 1c ). We emphasize that the burstiness and the fat tail effects are not necessarily related [46] . For instance, a power law ρ (Δ t ) ∝ (Δ t +1) −3 restricted to times Δ t ≤ T (sharp cutoff), is arbitrarily bursty but has no tail at all ( τ tail =0) for large but finite T . On the other hand, the delayed power law ρ (Δ t ) ∝ (Δ t − T ) −4 restricted to times Δ t ≥ T +1 has a fat tail (it decreases subexponentially, τ tail =∞) but low burstiness β for large T , as the mean time μ increases without bound and the variance remains constant. In the latter case, as for all pure power laws, ρ (Δ t ) ∼ Δ t − γ for large Δ t , the mixing time τ mix , as τ tail , is actually infinite, reflecting that mixing or relaxation to stationarity occurs only with subexponential convergence. In general, the properties of the tail of the distribution depend on the high-order moments of the distribution and not only on the first two moments as captured in the coefficient of burstiness. In Fig. 2 , we study the mechanism dominating the mixing time in toy synthetic temporal networks with different waiting-time distributions. Not surprisingly, structure is the driving mechanism when waiting times are narrowly distributed around a mean value, as in the case of Dirac (discrete time, Fig. 2c ) and Erlang distributions (resembling a discrete-time distribution with small fluctuations, Fig. 2d ). For those, the slowdown factor , comparing the exact mixing time (computed with equation (18) in Methods), with what it would be with memoryless waiting times , takes value in [0.6,1]. This indicates a limited speed up of the mixing due to negative burstiness, β <0, whereas the structure plays a major role through traversing orders of magnitude. 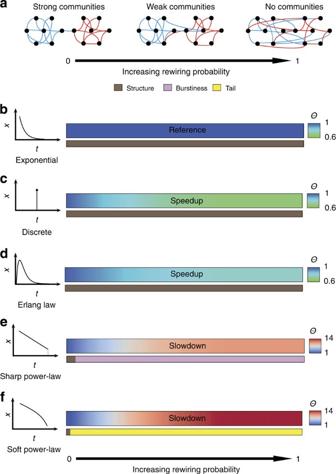Figure 2: Network structure or waiting times regulate mixing times. We illustrate the findings with a simple network composed of two communities, where the community structure is modulated by rewiring edges starting from two separated random graphs, as shown ina. Each panel (b–f) shows (on the top bar) for each value of the rewiring probability the slowdown factor Θ, ratio of the exact mixing time for a given waiting-time distribution and for the exponential case (Poisson process). Each panel corresponds to a different waiting-time distribution and the colourbar scale on the right represents the values of Θ for the respective colourmap. Θ close to one indicates that non-trivial waiting-time patterns can be neglected in the determination of the mixing time. On the other hand, a high Θ indicates that the details of the network structure are overshadowed by the temporal dynamics. (b) The reference case, that is, the exponential waiting times. We observe a speedup (Θ<1) for (c) Dirac (discrete) and (d) Erlang distributions, and a slowdown (Θ>1) for (e) a power law with sharp cutoff and for (f) a power law with soft cutoff. From left to right, we show how this factor depends on the network structure by progressively removing the community structure (increasing). The bottom bar of each panel shows, according to equation (14), which is the dominant factor, either structure, burstiness or tail, regulating the relaxation time for each model of waiting times. See Methods for details on the synthetic networks and waiting-time distributions. Figure 2: Network structure or waiting times regulate mixing times. We illustrate the findings with a simple network composed of two communities, where the community structure is modulated by rewiring edges starting from two separated random graphs, as shown in a . Each panel ( b – f ) shows (on the top bar) for each value of the rewiring probability the slowdown factor Θ, ratio of the exact mixing time for a given waiting-time distribution and for the exponential case (Poisson process). Each panel corresponds to a different waiting-time distribution and the colourbar scale on the right represents the values of Θ for the respective colourmap. Θ close to one indicates that non-trivial waiting-time patterns can be neglected in the determination of the mixing time. On the other hand, a high Θ indicates that the details of the network structure are overshadowed by the temporal dynamics. ( b ) The reference case, that is, the exponential waiting times. We observe a speedup (Θ<1) for ( c ) Dirac (discrete) and ( d ) Erlang distributions, and a slowdown (Θ>1) for ( e ) a power law with sharp cutoff and for ( f ) a power law with soft cutoff. From left to right, we show how this factor depends on the network structure by progressively removing the community structure (increasing ). The bottom bar of each panel shows, according to equation (14), which is the dominant factor, either structure, burstiness or tail, regulating the relaxation time for each model of waiting times. See Methods for details on the synthetic networks and waiting-time distributions. Full size image On the other hand, competition between structure and time appears in scenarios of high temporal heterogeneity. For example, only strong communities are able to dominate power-law waiting times ( Fig. 2e,f ). The effect of structure on the mixing times is otherwise removed as burstiness ( Fig. 2e ) or tail ( Fig. 2f ) becomes the leading mechanism, scaling the mixing times up to 14-fold in the shown configurations. The transitions between the different mechanisms for a range of power-law configurations are presented in Supplementary Fig. 1 and Supplementary Note 1 . Model reduction The use of coarse-graining through time-scale separation, which is the separate treatment of fast and slow dynamics that coexist inside a system, is crucial to reduce the complexity of systems made of a large number of interacting entities [50] , [51] , [52] . This procedure is well known for differential equations such as equation (2). In this case, it consists in neglecting fast decaying modes, for example, with decay time less than a certain threshold τ tresh —an approximation invalid for early times but acceptable for times significantly larger than τ tresh . Only the dominant modes, thus fewer variables, are left in the reduced model. Decreasing the threshold time, one produces a full hierarchy of increasingly more accurate models, but also with increasingly more variables. Reduced models have a clear interpretation from the structural point of view, as fast modes typically correspond to the fast convergence of the probabilities of the presence on nodes to a quasi-equilibrium within a network community. This process is followed by a slow equilibration of the population of random walkers trapped in each community to a global equilibrium [52] , [53] , [54] . Each new reduced variable can therefore be interpreted as the slow-varying probability of the presence in each community, as if it had been collapsed into a single node. The hierarchy of increasingly more accurate and complex reduced models corresponds in this structural picture to a hierarchy of increasingly finer partitions into communities. Given that the decay times of the different modes in equation (2) correspond to the Laplacian eigenvalues, the k -community partition is unsurprisingly found to be encoded into the k dominant Laplacian eigenvectors, in a way that is decoded by spectral clustering algorithms [55] , [56] . This methodology can be extended to a more general temporal operators D , where the successive decay times now depend on the Laplacian eigenvalues and the temporal characteristics following equation (13). However, the effect of temporality may have non-trivial consequences, as it may limit the number of reduced models. As an extreme scenario, let us consider a complex network in which the transient dynamics is dominated by the fat tail of the waiting-time distribution, such that all transient modes decay for large times as . Following equation (8), the approach to stationarity is described by the superposition of modes, all of the form , for various functions f k ( t ) that decay more slowly than exponentially, as for example . Among those, any mode can only become negligible with respect to another after a very long time. For all practical purposes, the system exhibits an inherently complex dynamics with no timescale separation, as the fine-scale structure (the finest being at the level of a single node) and the large-scale network communities have equal or similar impact on the random walk dynamics. As a consequence, only two reduced models are available, one in which all N modes are considered and another described solely by the stationary state. In general, only the Laplacian eigenvalues smaller in magnitude than μ / τ tail determine corresponding decay times. Just similar to that in classical memoryless case, they generate a hierarchy of timescales and reduced models corresponding to multiple levels of community structures. For instance, if five eigenvalues are smaller than μ / τ tail , thus 0= λ 0 > λ 1 > ⋯ > λ 4 >− μ / τ tail , then there is a reduced diffusion model capturing the movement of the random walker between five aggregated nodes. The mixing, internal to each community and decaying as , is considered instantaneous at large-enough timescales. Coarser aggregation, for example, based on two communities and two eigenvalues λ 0 , λ 1 , may be relevant, although valid only at even larger times. However, aggregation based on any finer partitioning (other than into one-node communities) has the same accuracy as the five-community model and thus little practical value as a reduced model. The degeneracy of characteristic decay times therefore limits the number of useful reduced models. This implies that a decomposition into communities is not necessarily associated to a timescale separation, or a reduced model, of the dynamics. For this reason, only models incorporating 1–5 or N -dominating modes are adequate for this particular example. This smaller choice of reduced models has ambivalent consequences. It limits the set of resolutions at which to describe the dynamics, but also provides a natural level for community structure (an open problem in multi-scale community detection [57] , [58] , [59] , [60] , [61] ), defined as the finest partitioning yielding a reduced model for the system. Numerical analysis Equation (14) shows that the mixing time depends in first approximation only on the mean, variance and tail of the waiting-time distribution, whereas other properties of the distribution are irrelevant. With numerical simulations, we validate this approximation and provide some quantitative intuition on the competition between the three factors regulating the mixing. We construct synthetic temporal networks respecting our assumptions, for example, stationarity or the absence of correlations and calibrate them with the static structure and the inter-contact time distribution observed on a number of empirical data sets. The empirical networks used for calibration correspond to face-to-face interactions between visitors in a museum (SPM), between conference attendees (SPC) [13] and between hospital staff (SPH) [16] ; email communication within a university (EMA) [10] ; sexual contacts between sex workers and their clients (SEX) [14] ; and communication between members of a dating site (POK) [12] (see Methods). On these networks, we observe the waiting-time distribution and the spectral gap, which allows to compute both the exact mixing time, with equation (18) in Methods, and its approximation in equation (14). The results, reported in Table 1 , show a good agreement, except for SPC, as analysed later in this section. Table 1 Exact versus approximate mixing times. Full size table Except for SEX [42] and POK data sets, in the other cases the temporal heterogeneity substantially increases the mixing times (see slowdown factor Θ in Table 1 ). Table 2 shows that in these networks the dominant factor regulating the mixing time depends on the characteristics of the system. Fat tails of the waiting-time distribution drive the relaxation for the cases of face-to-face contacts (SPM, SPC and SPH). However, the structure is the leading mechanism behind the networks corresponding to other situations of human communication (EMA, SEX and POK). Table 2 Dominating mechanisms on temporal networks. Full size table If communities are completely removed by randomizing the network structure, the link sparsity of SEX and POK networks guarantees that structure remains dominating, as the sparsity results in the inevitable creation of bottlenecks for diffusion even in a random network. On the other hand, in the EMA network, which has a relatively dense connected structure, the absence of communities leads to temporal dominance ( Table 2 ). Finally, when the contact times are uniformly distributed, we recover the well-known result that network structure, with or without communities ( Table 2 ), is the main factor regulating the convergence to stationarity. As the raw empirical temporal networks do not necessarily abide by our simplifying assumptions, one cannot validate our theoretical derivations, for example, by estimating the mixing time directly from simulations on empirical data. Indeed the periodic rythms or correlations between successive jumps or other temporal patterns may induce effects not captured by our formula, as discussed in Supplementary Table 1 and Supplementary Note 3 . Empirical data are collected during a finite time span T , leaving the choice between a model for ρ (Δ t ) that is limited to T (sharp cutoff) or extrapolated to infinite times with a tail decay (soft cutoff). The latter may occur, for instance, if we have theoretical or practical reasons to prefer a fat-tail-based model (for instance power law) with exponential cutoff for ρ (Δ t ). This choice is of little impact on the results, provided a sufficient observation time T ( Supplementary Note 2 ). When temporal patterns trump structure, we have a self consistency condition ( Table 2 ) for SPM and SPH, expressing that both models lead to similar mixing times, albeit through the different mechanisms of either burstiness (sharp) or fat tail (soft). For SPC, self-consistency is not attained. This happens possibly because the observation time of ∼ 2 days is not sufficiently large to dilute the irregularity on the observed inter-contact time distribution (thus, in the simulated waiting times) induced by the inactivity during night periods. Consequently, this makes the tail difficult to measure, as it has not clearly emerged from a still transient behaviour, and a significant mismatch is observed between exact and approximate mixing ( Table 2 ). We evaluate the possible sizes of reduced models for the data as follows. As the eigenvalues λ k of the Laplacian range between 0 and −2, the number of modes with structurally determined decay times (− μ / τ tail < λ k ≤0) can be roughly evaluated to Nμ /2 τ tail on an N -node network, if eigenvalues are evenly spaced. A similar reasoning holds whenever burstiness dominates the tail effect. This analysis reveals three different scenarios in the structure-dominated data sets considered above: (i) SEX benefits from a full hierarchy of reduced models, as μ /2 τ tail >1. (ii) The dynamics on EMA can be approximated with just three modes, associated to three network communities, as 0= λ 0 > λ 1 > λ 2 >− μ / τ tail > λ 3 >…, while a more detailed description, unless at the node level, would not gain any significant accuracy as further modes are all degenerate with the same decay time μ / τ tail . (iii) POK exhibits a practically full hierarchy of reduced models, as around one third of its modes are determined by structure, μ /2 τ tail =0.33; therefore, the finest reduced model is at a few-node community level. This spectral analysis is comforted by applying a multiscale community detection algorithm to the empirical networks, which finds a partition into three communities dominated by fat-tail effects for EMA, but not for POK or SEX ( Fig. 3 ). 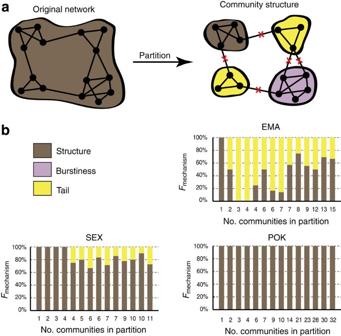Figure 3: Global mixing time versus mixing times in communities. (a) Although the mixing time of diffusion on a network may be defined by the community structure, diffusion in the communities themselves may be regulated by structural or temporal patterns. (b) The original network constructed from an empirical data set is divided into communities with a multi-resolution community detection algorithm, for different values of the resolution parameter (see Methods). For each partition, we identify the fraction of communities with more than 10 nodes (yaxis), where either structure or tail dominates (according to equation (14)), and plot against the number of communities detected at each partition (xaxis). This confirms our spectral analysis, which predicts a compact description of the diffusion dynamics on EMA into three modes describing a probability flow between three communities, each dominated by fat-tailed waiting times. Also in agreement with the spectral viewpoint, this is not the case for SEX or POK, unless at the level of a few-node communities. Figure 3: Global mixing time versus mixing times in communities. ( a ) Although the mixing time of diffusion on a network may be defined by the community structure, diffusion in the communities themselves may be regulated by structural or temporal patterns. ( b ) The original network constructed from an empirical data set is divided into communities with a multi-resolution community detection algorithm, for different values of the resolution parameter (see Methods). For each partition, we identify the fraction of communities with more than 10 nodes ( y axis), where either structure or tail dominates (according to equation (14)), and plot against the number of communities detected at each partition ( x axis). This confirms our spectral analysis, which predicts a compact description of the diffusion dynamics on EMA into three modes describing a probability flow between three communities, each dominated by fat-tailed waiting times. Also in agreement with the spectral viewpoint, this is not the case for SEX or POK, unless at the level of a few-node communities. Full size image We have presented a unified mathematical framework to calculate the relaxation time to equilibrium in a wide variety of stochastic processes on networked temporal systems. Our formalism is able to refer to arbitrary linear multi-agent complex systems, including linearizations of non-linear dynamical models such as Kuramoto oscillators or non-Laplacian diffusion dynamics such as Susceptible-Infected-Recovered epidemics, as detailed in Methods. It is also possible to accommodate non-uniformity of parameters as nodes are not identical in real systems. Our results are particularly relevant to improve the understanding of temporal networks, by highlighting the important interplay between structure and the temporal statistics of the network. Our formalism is different from previous studies of random walks on temporal networks that focus on homogeneous temporal patterns [23] or do not account for the competition between structure and time [15] . We emphasize that questions related to ordering, not timing of events, such as the number of hops before stationarity or the succession of nodes most probably traversed by the walker, depend on the structure alone and not of hops timing statistics. Moreover, key mechanisms have been left aside in our modelling approach, such as the non-stationarity or periodicity of most empirical networks [19] , [20] , [21] and the existence of correlations between edge activations, and therefore preferred pathways of diffusion [17] , [18] , [41] . Important future work includes their incorporation in our mathematical framework and the identification of dominant mechanisms in empirical data. We have shown that in the absence of some temporal correlations, the characteristic times of the dynamics are dominated either by temporal or by structural heterogeneities, as those observed in real-life systems. The competing factors are not only observed in different classes of networks modelled from empirical data but also at different hierarchical levels of the same network represented by its different scales of community structure. We have also identified two contrasting metrics of the statistics of waiting times, burstiness and fat tails. We have shown that they regulate the dynamics on the network in different ways. In systems where temporal patterns are the dominating factor, the reduced models obtained by aggregation of communities as commonly used in practice are not necessarily relevant, as small-scale details are impenetrably intertwined with large-scale structure to form a complex global dynamics. In general, the temporal characteristics impose the natural description levels of the dynamics. Altogether, our results suggest the need for a critical assessment of a complexity/accuracy trade-off when modelling network dynamics. In some classes of real-world systems, the burden of increased model complexity may not compensate the incremental gain in knowledge, whereas other systems require the fine network structure as a key ingredient to any realistic modelling. Overview We provide a description of multi-agent linear dynamics, detail the derivation of approximation (12) and its range of validity, illustrate the generality of the framework beyond random walks and describe the empirical data and numerical implementations. In the Supplementary Information , we discuss on power laws and cut offs ( Supplementary Note 1 and Supplementary Fig. 1 ), the evaluation of waiting-time distributions in empirical data ( Supplementary Note 2 ) and the adequacy of our theoretical framework in empirical networks with correlations and non-stationarity ( Supplementary Note 3 ). Linear multi-agent systems We derive equation (1) for general linear-networked systems, or multi-agent systems [30] , with an illustration on consensus dynamics. Every node i is modelled by a linear agent whose internal state is initially zero, and that converts an input signal u i with an operator F i —the so-called transfer function—into a state signal x i = F i u i . Here, u i represents a time trajectory u i ( t ) or its Laplace transform u i ( s ), and similarly for the state trajectory x i . The transfer function F i is an operator mapping input trajectories u i to state trajectories x i , which is requested to be linear, causal (if u i ( t )=0 for all t < T , then the same holds for x i ( t )) and time invariant (shifting u i ( t ) in time results in shifting x i ( t )). Under those conditions, this operator takes the form x i ( s )= F i ( s ) u i ( s ), a simple product of functions, in the Laplace domain. When using Laplace transforms, it is customary to use time domain trajectories that are zero for negative times. We account for the state initial condition x i (0)= x i ,0 with another input term v i that can be, for example, an impulse exciting the rest state to any desired initial condition at time zero. The agent dynamics therefore writes x i ( s )= F i ( s )( u i ( s )+ v i ( s )). For instance if F i is the integration operator in the time domain, from the initial value at time 0, or in other terms (for the Dirac impulse δ ( t )), then in the Laplace domain we find x i ( s )=1/ s ( u i ( s )+ x i ,0 ); in this case, the Laplace domain operator is the multiplication by 1/ s and v i is a Dirac impulse in the time domain, a constant in the Laplace domain that encodes the initial condition. One can as well invert the transfer operator, , and write d x i /d t = u i ( t )+ x i ,0 δ ( t ) or sx i ( s )= u i ( s )+ x i ,0 ; here, the Dirac impulse is seen as arising from differentiating the discontinuous step of the state from rest to initial condition x i ,0 . Connecting agents such that the input u i ( t ) of agent i is a weighted sum of other agents’ states, Σ j L ij x j ( t ) leads to a global dynamics d x /d t = L x + x 0 δ ( t ), or equivalently s x ( s )= L x ( s )+ x 0 , where L is the matrix of entries L ij , x is the vector of states x i and x 0 is the vector of initial conditions x i ,0 . When L is a Laplacian (rows summing to zero, non-negative off-diagonal weights), this is a simple consensus system where agents (for instance, robots or individuals) change their state (for instance, position, opinion modelled as a real number) towards an average of their neighbours’ states. With arbitrary interconnection weights and arbitrary transfer functions, one similarly obtains where D is the diagonal matrix of transfer functions ( D reduces to a scalar in case of identical agents F i = F j ) and v the vector of initial condition input v i . The case when L remains Laplacian, but D is arbitrary, describes general, higher-order consensus systems where the agents converge to equal values on a strongly connected network through arbitrarily complicated internal dynamics, for example, modelling realistic robots or vehicles. For example, vehicles of mass m driven by a force and friction will obey . An abuse of notation allows to drop implicitly the initial condition and write simply dx/d t = L x and more generally equation (1), D x= L x, instead of equation (15) above. Discrete-time systems are recovered with a discrete-derivative operator D x( t )=x( t +1)−x( t ). Exact and approximate characteristic times for random walkers We derive the approximate characteristic times (equation (12)) of decaying modes associated to a general random walk. The dominant mode associated to λ 0 =0 is the stationary distribution, unique for an ergodic random walk. The relaxation time to the stationary distribution, generalizing the well-known mixing time of Markov chain theory [36] , is the characteristic time of the slowest decaying mode after the stationary mode, usually associated to λ 1 , as we suppose here. An example of a case when λ 1 is not associated to the mixing mode, but rather λ N , is the discrete random walk, where the distribution is a Dirac distribution at μ , with zero variance, and the network is bipartite or close to bipartite. The characteristic decay time of a time-domain function can be found in the Laplace domain, as f ( s ) is defined and analytic over all s of real part larger than −1/ τ decay , but undefined or non-analytic in at least one point s of real part−1/ τ decay . For example, the Laplace transform of is 1/(1+ τ decay s ), with pole at s =−1/ τ decay , and the Laplace transform of for γ >1 is defined, but is non-analytic at s =−1/ τ decay . The eigenfunction z k ( t ) associated to λ k is the solution of D ( s ) z k ( s )= λ k z k ( s )+ D ( s ) z k ( t =0)/ s , derived in the text as equation (6), with D ( s )=1/ ρ ( s )−1 and L replaced with λ k . The decay time of z k ( t ) is found if we find the right-most non-analytic point of derived in the main text as equation (9). Note that for λ k ≠0, the singularity in s =0 is only apparent as D ( s )= μs −( σ 2 − μ 2 ) s 2 /2+… This expression is non-analytic in s in exactly two circumstances: (i) D ( s ) is non-meromorphic in s , meaning that it cannot be defined analytically in a punctured neighbourhood of s (a neighbourhood of s − s ) or (ii) D ( s )= λ k . Case (i) happens when ρ ( s ) is non-meromorphic in s . A typical example is when , where ρ 0 ( t ) is a fat-tailed distribution, in other words decreases more slowly than any exponential, leading to a non-meromorphic transfer function—a rare occurrence in standard systems theory. The non-analytic point is precisely s =−1/ τ tail . Case (ii) commands to solve the equation whose solution s k enters the expression for the exact characteristic decay time, combining the two cases: which can be approximated from an expansion of ρ ( s ). It is noteworthy that ρ ( s )=1− μs +( μ 2 + σ 2 ) s 2 /2− ⋯ is also called the moment-generating function, whose successive derivatives around s =0 are the moments of the distribution, up to sign. We consider the Padé (that is, rational) approximation: equivalent for small s to a second-order Taylor approximation in terms of accuracy. This approximates the transfer function D −1 ( s )= F ( s )= ρ ( s )/(1− ρ ( s )) as where the adimensional term takes its minimum value at −1/2 for the discrete-time random walk, zero for a memoryless process and arbitrary large values for highly heterogeneous distributions. It is therefore a suitable measure of the burstiness of the process [41] , [47] . Such a transfer function is called Proportional-Integral, a common class in systems theory [29] . The equation D ( s )= λ k is approximately solved by 1/ s k ≈ μ (| λ k | −1 + β ). A possible non-analytic point at s =−1/ τ tail caps the characteristic decay time of eigenfunction k to If λ k −1 and β are of different orders of magnitude, one may further approximate as in which the influence of the fat tail, the structure and the burstiness are decoupled. The mixing time is associated with λ 1 . 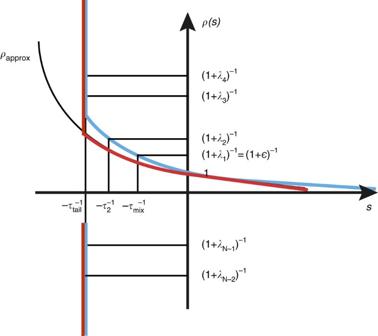Figure 4: The exact and approximate characteristic times of a waiting-time probability distribution. Computation of the characteristic time of the distribution(blue curve) with a fat-tailedρ0and a non-analytic point ats=−1/τtail.The exact characteristic decay timesτkare found from the eigenvalues and the blue curve, following equation (18). In this example, only three modes, including the stationary, are influenced by the structure of the network, whereas the other modes collapse to a single decay timeτtail. The dynamics can thus be approximated by three modes, typically describing aggregate probability flows between three network communities. The approximate solution equation (12) follows the red curve, constructed from the Padé approximantρapprox, see equation (19). As eigenvaluesλkchange from 0 to −2, the values 1/(1+λk) can take any real value >1 or <−1. Figure 4 shows that typically half of the modes have structurally determined decay times, namely those with positive 1+ λ k , if eigenvalues are uniformly spaced between 0 and −2, in apparent contradiction with the back of the envelope calculation Nμ /2 τ tail proposed in the main text, which can reach N . This is a consequence of the progressive degradation of the Padé approximation for larger s (larger eigenvalues). Figure 4: The exact and approximate characteristic times of a waiting-time probability distribution. Computation of the characteristic time of the distribution (blue curve) with a fat-tailed ρ 0 and a non-analytic point at s =−1/ τ tail. The exact characteristic decay times τ k are found from the eigenvalues and the blue curve, following equation (18). In this example, only three modes, including the stationary, are influenced by the structure of the network, whereas the other modes collapse to a single decay time τ tail . The dynamics can thus be approximated by three modes, typically describing aggregate probability flows between three network communities. The approximate solution equation (12) follows the red curve, constructed from the Padé approximant ρ approx , see equation (19). As eigenvalues λ k change from 0 to −2, the values 1/(1+ λ k ) can take any real value >1 or <−1. Full size image Even for small eigenvalues, for example, for , the approximation (equation (12)), thus also equation (14), has a limited range of validity. The underlying Padé approximation (equation (19)) is valid for small-enough s , while for large-enough s the exact solution is τ tail . The small s behaviour is captured by the first and second moments, and the large s behaviour, in other terms the tail τ tail , determines the growth of high-order moments. This double approximation based on high and low moments may explain why the approximation is successful on diverse data sets (see Fig. 3a ). However, it is likely to fail precisely when the intermediate moments (third, fourth and so on), not covered by the approximation, dominate the behaviour of the moment generating function ρ ( s ). This occurs for instance in the case of a power law of exponent >3 with sharp cutoff at a large time: although the first and second moment remain bounded and the tail is absent, the intermediate moments grow without bound with the cutoff time. However, such distributions are rarely used as models for real-life data. On the other hand, numerical experiments showed excellent accuracy for a wide range of power laws with soft cutoff. Beyond random walks Random walks are many times formally identical to the asymptotic behaviour of non-linear dynamical models and also serve as a prototype for a wider class of dynamics that includes epidemic spreading. For example, power networks may be modelled as a network of second-order Kuramoto oscillators [33] whose state in every node is a phase (an angle) θ i influenced by its neighbours where I is the inertia, α the friction and ω describes the natural frequency of the oscillation. In this construction, we assume identical parameters for each node. After the change of variables φ i = θ i − ωt / α , the linearization around the synchronized equilibrium ( φ i = φ j is constant for all times) is written which is formally identical to a consensus equation structured by the Laplacian L [33] . Hence, it supports the same formalism as random walks, after the operator D is changed accordingly. The linear dynamics associated to the asymptotic behaviour is often a crucial first step in understanding the non-linear dynamics of the network at some time scale. Another class of dynamical systems where our results apply are linear dynamics given by equation (1), but where the interaction matrix L does not have a Laplacian structure and where the dominant eigenmode is not necessarily stationary. This is the case, for instance, for epidemic processes where infected individuals diffuse on a meta-population network, where nodes are large populations (cities and so on), and the individuals may either reproduce (by contamination of a healthy individual) or die (or recover). One classic model for this process is a multi-type branching process. This is akin to a random walk whose number of walkers is not preserved in time, as random events are not limited to hops but also death or split. This kind of model also emerges as the linearization of classic compartmental epidemic models such as Susceptible-Infected or Susceptible-Infected-Recovered [62] . The waiting time between two consecutive events may also be described by an arbitrary distribution ρ (Δ t ). The expected number of walkers in time may again be described by an equation D x= L x, where D depends on ρ in the same way as before, but now L is no more a Laplacian and in particular may have negative and positive eigenvalues. If the epidemics is supercritical, then the system is unstable. This implies the existence of unstable eigenmodes ( λ k >0) where the number of walkers grow exponentially as , with τ k now approximated by . In this case, the fat tail of the waiting-time distribution does not play any role for the unstable eigenmodes. From this formula, we see that although the decay of stable eigenmodes tends to slow down due to burstiness and possibly fat tail, the unstable eigenmodes are boosted by burstiness. As a consequence, it leads in all eigenmodes to a long-term increase of the infected population due to the temporal heterogeneity. Numerical analysis We use six data sets of empirical networks: SPM, SPC [13] and SPH [16] ; EMA [10] ; SEX [14] ; and POK [12] (see Table 3 ). Table 3 Summary statistics of the empirical networks. Full size table The synthetic networks used in Fig. 2 are formed by 1,000 nodes and 10,000 links equally divided into two groups, initially disconnected (rewiring probability equal to zero). Within each group, pairs of nodes are formed between uniformly chosen nodes. A fraction of links are rewired to weaken communities. Rewiring consists of uniformly choosing two pairs of nodes and swapping the pairs. Rewiring probability equal to 1 removes any significant community structure from the network. Communities refer to groups of nodes with more connections between themselves than with nodes at other groups. The spectral gap is calculated for each network configuration. The exemplified waiting-time distribution are ρ (Δ t )=exp(−Δ t / μ )/ μ with μ =1 (exponential); =1.0 (discrete); ∝ Δ t k −1 exp(− k Δ t / μ ) with k =3 and μ =3 (Erlang law); ∝ Δ t − γ with γ =2 and cutoff at T =1,000 (power law with sharp cutoff); ∝ Δ t − γ exp(−Δ t / τ tail ) with γ =3 and τ tail =20 (power law with soft cutoff). The synthetic temporal networks used in Table 2 and Fig. 3 are constructed by using the unweighted version of the empirical networks as underlying fixed structures. The randomized networks used in Table 2 are obtained by uniformly selecting two pairs of nodes of the original network and then swapping the respective contacts. In the dynamic network, a node and its links alternate between inactive and active states. To fit this synthetic temporal network to our theoretical assumptions, we assume that all links of a node are activated simultaneously, the system is time invariant (no daily or weekly cycles), exhibits no temporal correlations between successive jumps and node-activation times are sampled from the same distribution of interactivation times (node homogeneity). The active state of a node and its links lasts for one time step δt , and then the node and links return to the inactive state. The distribution of interactivation times (a.k.a. inter-contact times) corresponding to the original times is obtained by pooling the times between two subsequent activations of the same node, in other words two consecutive contacts established between the node and its neighbourhood, as observed in the empirical networks [20] , [42] . The randomized times in Table 2 correspond to activation times sampled from exponential distributions with the same mean as the corresponding empirical cases. To obtain the waiting-time estimates presented in Table 2 , we simulate a random walk in these synthetic networks. A random walker starts in a randomly chosen node. As time goes by, a walker remains in the node until its new activation and then hops to a uniformly chosen neighbour. The waiting time is thus the time elapsed between the arrival and departure of the walker in a node. We simulate a single random walker and let it hop 300,000 times, starting at 10 uniformly chosen nodes; hence, we collect a total of 3 million points for the statistics of waiting times. Besides that, for each starting configuration we discard the initial 5,000 hops to remove the stochastic transient. The waiting-time distribution observed in the simulations provides us with estimates of τ mix , μ , σ 2 and τ tail . The mixing time τ mix is estimated from the distribution expressed in the Laplace domain through equation (18) (for k =1, the mixing mode). This equation is exact, as the synthetic data has been constructed so as to satisfy the conditions of validity under which it is proved. One could also estimate the mixing time from the convergence of random trajectories starting in a definite node towards stationarity; however, this exercise is computationally demanding. The exponential tail decay time τ tail is estimated using least-square fitting by a line in a lin-log plot of the second half of the waiting-time distribution data, thus between T max /2 and T max , where T max is the largest observed waiting time. Indeed, an exponential decay translates into a straight line in a lin-log plot, the slope of which determines the decay time. The choice of the interval [ T max /2, T max ] to perform a linear fit is steered by the want for a simple criterion uniform across data sets. This may be inappropriate for data sets where the observation time forces a cutoff on the data sets before the tail decay has had time to emerge, for instance in SPC, where a more careful definition of tail, for example, on a smaller interval, may be more adequate. Let us interpret some elementary observations that can be made on Table 2 . From (a) to (b), τ tail is only approximately preserved, because it is recomputed from the simulated waiting-time distribution on a different network, thus a slightly different distribution, even though the inter-contact times are sampled from the same distribution in both panels. In (c) and (d), the inter-contact time distribution is memoryless (exponential), thus identical to the waiting-time distribution regardless of the network, and τ tail coincides with μ . From (a) to (c), the quantity drops sharply, although is clearly preserved as the network is unaltered. The reason is that although the mean inter-contact time is preserved by construction, the mean waiting time also depends on the variance of the inter-contact times, in virtue of the bus paradox, and this variance is clearly strongly affected by the time randomization. The drop in from (b) to (d) is associated to the same mechanism. To identify the community structure of the empirical networks in Fig. 3 , we use the partition stability method [54] using a freely available implementation [63] . The method uses a simple diffusion process such that different communities are detected at different time scales according to the potential of the communities to trap the diffusion at the given time scale. Optimal communities have been derived for values of the resolution parameter decreasing from 10 2 ,10 1.95 ,10 1.9 ,10 1.85 ,…, with increasingly fine partitions. After identifying the relevant communities, we discard the inter-community links and calculate the spectral gap of each individual community of at least ten nodes. How to cite this article: Delvenne, J.-C. et al . Diffusion on networked systems is a question of time or structure. Nat. Commun . 6:7366 doi: 10.1038/ncomms8366 (2015).